The smooth muscle-selective RhoGAP GRAF3 is a critical regulator of vascular tone and hypertension Although hypertension is a worldwide health issue, an incomplete understanding of its aetiology has hindered our ability to treat this complex disease. Here we identify arhgap42 (also known as GRAF3) as a Rho-specific GAP expressed specifically in smooth muscle cells (SMCs) in mice and humans. We show that GRAF3-deficient mice exhibit significant hypertension and increased pressor responses to angiotensin II and endothelin-1; these effects are prevented by treatment with the Rho-kinase inhibitor, Y27632. RhoA activity and myosin light chain phosphorylation are elevated in GRAF3-depleted SMCs in vitro and in vivo , and isolated vessel segments from GRAF3-deficient mice show increased contractility. Taken together, our data indicate that GRAF3-mediated inhibition of RhoA activity in vascular SMCs is necessary for maintaining normal blood pressure homoeostasis. Moreover, these findings provide a potential mechanism for a hypertensive locus recently identified within arhgap42 and provide a foundation for the future development of innovative hypertension therapies. Although hypertension is a major risk factor for stroke, myocardial infarction and kidney failure, we know surprisingly little about the pathophysiology of its development. One reason for this is that blood pressure is a complex trait that is regulated by many organ systems and a large number of humoral factors. Increased peripheral vascular resistance due to decreased arteriolar vessel diameter is a common feature of hypertension. This parameter is controlled, at least in part, by the contraction of vascular smooth muscle cells (SMCs) within the resistance arterioles [1] , [2] , [3] , [4] , [5] and many antihypertensive therapies inhibit the signalling pathways that control SMC contractility. In contrast to skeletal and cardiac muscle, excitation–contraction coupling in SMC is mediated by the Ca 2+ -dependent activation of myosin light chain kinase, and SMC tension is directly proportional to myosin light chain (MLC) phosphorylation [6] , [7] . SMC contractility is also enhanced by activation of the small GTPase RhoA, which leads to Rho-kinase (ROCK)-dependent inhibition of myosin phosphatase [8] , [9] , [10] , [11] . Many GPCR-coupled contractile agonists including angiotensin II (AngII), norepinephrine, endothelin-1 (ET-1), stimulate RhoA in SMC, and several lines of evidence have implicated RhoA signalling in the development of hypertension. Increased ROCK activity has been observed in spontaneously hypertensive rats and some hypertensive patient populations [8] , [12] and ROCK inhibitors like Y27632, Fasudil and SAR407899 have been shown to reduce blood pressure in hypertensive animal models and patients [13] . Recent studies in genetically modified mice demonstrated that germline deletion of the Rho-specific guanine exchange factor (GEF), LARG, inhibited salt-induced hypertension [14] whereas SMC-specific knockout of the related GEF, p115RhoGEF, inhibited the development of hypertension in response to AngII [12] . RhoA activity is limited by GAPs that facilitate RhoA’s intrinsic GTPase activity, but little is known about the involvement of RhoGAPs in the regulation of SMC contractility or the development of hypertension. Several recent genome-wide association studies have identified novel genetic polymorphisms that contribute to variations in blood pressure and other cardiovascular disease end-points [15] . Most of these are found within or near genes that have no known connection to the control of blood pressure, and a critical next step is to determine the mechanism by which they exert their effects. One such locus on chromosome 11 represented by SNPs rs633185 and rs604723 is within the 80 KB first intron of FLJ32810 (refs 16 , 17 ). This gene, which was later annotated as arhgap42 (also known as GRAF3), is a member of the GRAF family of Rho-specific GAPs whose founding member, GRAF1, was originally described by our group [18] , [19] , [20] . Although we showed that GRAF1 plays an important role in limiting RhoA activity in terminally differentiated cells (that is, skeletal muscle, heart and brain), no studies to date have explored the expression or function of GRAF3 (refs 19 , 20 , 21 ). Interestingly, our genome-wide analyses of chromatin structure in primary human SMC by DNAse hypersensitivity identified several regions within the GRAF3 gene that were selectively ‘open’ in SMC compared with over 25 other human cell types, suggesting that this gene was regulated in a smooth muscle-specific fashion (C.M., personal communication). Given the known involvement of RhoA and RhoGEFs in the control of blood pressure, we hypothesized that GRAF3’s association with blood pressure regulation was mediated by its ability to inhibit RhoA in SMC. Herein we validate GRAF3 as a Rho-specific GAP and show that it is strongly and specifically expressed in SMC. Importantly, we found that GRAF3-deficient mice are significantly hypertensive and exhibit ROCK-dependent increases in contractile agonist-induced pressor responses. Collectively, these data indicate that GRAF3-dependent inhibition of RhoA activity in vascular SMC is necessary for maintaining normal blood pressure homoeostasis. GRAF3 is expressed in a smooth muscle-restricted fashion Immunohistochemical analysis of mouse and human tissues with two distinct GRAF3 antibodies that do not react with GRAF1 or GRAF2 ( Supplementary Fig. S1a,b ), revealed that GRAF3 was highly and selectively expressed in SMC ( Fig. 1 ; Supplementary Figs S1c and S2d,e ). As shown by co-staining with SM α-actin and PECAM, GRAF3 expression was limited to the medial SMC layer in all vessels and to the SMC layers of the stomach, intestine and lung. Reverse transcription polymerase chain reaction (RT–PCR) confirmed that GRAF3 RNA was highly abundant in primary SMC isolated from rodent aortae and in GI tissues that contain a large SMC component (see Figs 2b and 4b ; Supplementary Fig. S2b,c ). 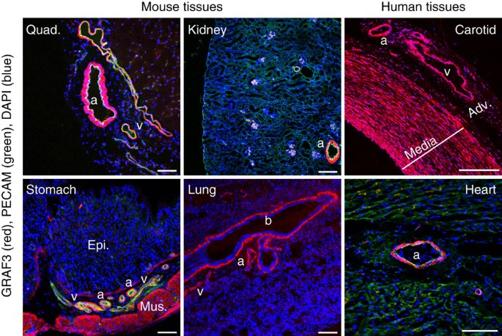Figure 1: GRAF3 is expressed in a smooth muscle-restricted fashion. Tissues from Wt mice (2–14-week-old) or human (2 years) were frozen in OCT, sectioned and stained with a specific GRAF3 antibody (red; also seeSupplementary Fig. S1andSupplementary Fig. S2d,e). Some samples were co-stained with PECAM antibody (green). DAPI is shown in blue. a, arteriole/artery; b, bronchi; v, vein; adv., adventitia; Epi., epithelial layer; Mus., smooth muscle layer. Note strong expression of GRAF3 throughout the media of human carotid artery and in the microvessels within the adventitia. Scale bars, 100 microns for mouse tissue and 550 microns for human tissues. Figure 1: GRAF3 is expressed in a smooth muscle-restricted fashion. Tissues from Wt mice (2–14-week-old) or human (2 years) were frozen in OCT, sectioned and stained with a specific GRAF3 antibody (red; also see Supplementary Fig. S1 and Supplementary Fig. S2d,e ). Some samples were co-stained with PECAM antibody (green). DAPI is shown in blue. a, arteriole/artery; b, bronchi; v, vein; adv., adventitia; Epi., epithelial layer; Mus., smooth muscle layer. Note strong expression of GRAF3 throughout the media of human carotid artery and in the microvessels within the adventitia. Scale bars, 100 microns for mouse tissue and 550 microns for human tissues. 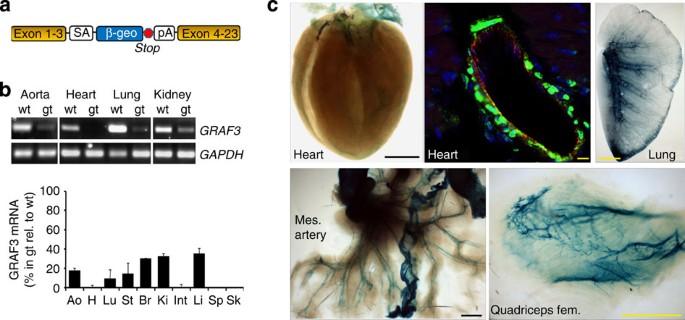Figure 2: Development of GRAF3 hypomorphic mice. (a) Schematic of gene trap insertion site in the SIGTR CE0477 ES clone. 5′ RACE revealed the gene trap cassette (β-geo) was located in intron 3 (seeSupplementary Table S1), and this locus was verified and further refined using a targeted PCR approach that revealed the site of integration between chromosome 9: 9,082,984–9,083,121 (reverse strand). (b) RT–PCR analysis of GRAF3 (exon 1–4) and GAPDH mRNA levels in tissues from Wt and GRAF3gt/gtmice (quantification shown graphically below; mean±s.e.m.,n=3/genotype). Similar results were found using primers to target downstream exons (seeSupplementary Fig. S2b). (c) GRAF3 expression pattern revealed by whole mount Lac Z staining (blue; scale bars, 1.5 mm) or by dual immunohistochemical staining for β-GAL (green; scale bar, 10 microns), PECAM (red), (DAPI, blue) in frozen sections (coronary vessel, top–middle) from GRAF3+/gtmice. Vessel-restricted LacZ staining was also evident in brain (seeSupplementary Fig. S2f). No significant LacZ staining or β-GAL immunofluorescence was observed in tissues from Wt mice.Mes., mesenteric. Full size image Figure 2: Development of GRAF3 hypomorphic mice. ( a ) Schematic of gene trap insertion site in the SIGTR CE0477 ES clone. 5′ RACE revealed the gene trap cassette (β-geo) was located in intron 3 (see Supplementary Table S1 ), and this locus was verified and further refined using a targeted PCR approach that revealed the site of integration between chromosome 9: 9,082,984–9,083,121 (reverse strand). ( b ) RT–PCR analysis of GRAF3 (exon 1–4) and GAPDH mRNA levels in tissues from Wt and GRAF3 gt/gt mice (quantification shown graphically below; mean±s.e.m., n =3/genotype). Similar results were found using primers to target downstream exons (see Supplementary Fig. S2b ). ( c ) GRAF3 expression pattern revealed by whole mount Lac Z staining (blue; scale bars, 1.5 mm) or by dual immunohistochemical staining for β-GAL (green; scale bar, 10 microns), PECAM (red), (DAPI, blue) in frozen sections (coronary vessel, top–middle) from GRAF3 +/gt mice. Vessel-restricted LacZ staining was also evident in brain (see Supplementary Fig. S2f ). No significant LacZ staining or β-GAL immunofluorescence was observed in tissues from Wt mice. Mes. , mesenteric. Full size image Figure 4: GRAF3 depletion in cultured SMC promotes Rho activity. 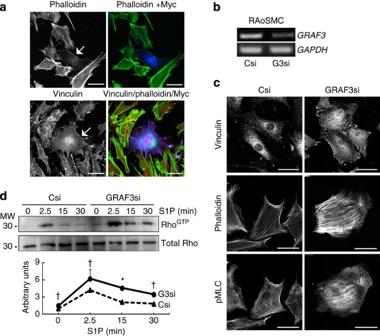Figure 4: GRAF3 depletion in cultured SMC promotes Rho activity. (a) Ectopic expression of myc-GRAF3 (arrow, left; blue, right) in rat aortic SMC (RAoSMC) induced marked clearing of actin stress fibres as assessed by phalloidin staining (white, left or green, right) and focal adhesions as marked by vinculin (white, left or red, right). (b) Levels of GRAF3 and GAPDH mRNA in control (Csi) and GRAF3 (G3) si-treated RAoSMC. Data are representative of seven separate experiments. (c) GRAF3 si-treated RAoSMC exhibited a more contractile morphology (more abundant vinculin-labeled focal adhesions and phalloidin-labeled stress fibres) and elevated phospho-MLC (pMLC) when compared with control si (Csi)-treated cells. Scale bars for panelsaandcare 50 microns. (d) GRAF3 si and Csi-treated RAoSMC were stimulated with S1P and active (GTP-bound) RhoA was precipitated with GST-rhotekin beads and assessed by immunoblotting (top panel). Densitometric analysis of three separate experiments is presented as mean±s.e.m. (bottom panel).Pvalues (Student’st-test) are expressed as: †P<0.1; *P<0.05. ( a ) Ectopic expression of myc-GRAF3 (arrow, left; blue, right) in rat aortic SMC (RAoSMC) induced marked clearing of actin stress fibres as assessed by phalloidin staining (white, left or green, right) and focal adhesions as marked by vinculin (white, left or red, right). ( b ) Levels of GRAF3 and GAPDH mRNA in control (Csi) and GRAF3 (G3) si-treated RAoSMC. Data are representative of seven separate experiments. ( c ) GRAF3 si-treated RAoSMC exhibited a more contractile morphology (more abundant vinculin-labeled focal adhesions and phalloidin-labeled stress fibres) and elevated phospho-MLC (pMLC) when compared with control si (Csi)-treated cells. Scale bars for panels a and c are 50 microns. ( d ) GRAF3 si and Csi-treated RAoSMC were stimulated with S1P and active (GTP-bound) RhoA was precipitated with GST-rhotekin beads and assessed by immunoblotting (top panel). Densitometric analysis of three separate experiments is presented as mean±s.e.m. (bottom panel). P values (Student’s t -test) are expressed as: † P <0.1; * P <0.05. Full size image Development of GRAF3 hypomorphic mice To explore GRAF3’s role in regulating vessel tone and blood pressure homoeostasis in vivo , we generated a GRAF3-deficient mouse line using ES cells that contained an inhibitory LacZ gene tap within the GRAF3 third intron ( Fig. 2a , Supplementary Fig. S2a and Supplementary Table S1 ). Crosses between GRAF3 +/gt mice yielded offspring in the appropriate Mendelian ratios, and no overt phenotypes were observed in GRAF3 +/gt or GRAF3 gt/gt mice for up to 6 months ( Supplementary Table S2 ). GRAF3 message was strongly but not completely depleted in all tissues evaluated indicating that our gene trap model results in a hypomorphic allele ( Fig. 2b , Supplementary Fig. S2c ). Importantly, GRAF3 messenger RNA (mRNA) levels in the aorta and coronary vasculature were reduced by 80% and 99%, respectively and reductions in GRAF3 message were consistent in all tissues at all time points analysed (between 2 and 16 weeks postnatal). Tissue-specific differences in residual GRAF3 mRNA levels in our model were likely due to the differential expression or activity of splicing factors [22] . Inclusion of the LacZ/neo insertion cassette into the GRAF3 transcript results in a heterologous protein that contains GRAF3 amino acids 1-104 fused in frame to the β-Gal reporter gene ( Fig. 2a ). As expected, β-Gal staining in gene trap mice closely mimicked endogenous GRAF3 expression with strong and selective staining within the heart, mesenteric, skeletal muscle and brain arterioles and the SMC layers of the GI tract ( Fig. 2c , Supplementary Fig. S2f ). High power images co-stained with β-Gal and PECAM antibodies revealed that expression in the vasculature including coronary and renal vessels was restricted to SMC. GRAF3 depletion elevates vessel tone and blood pressure We evaluated blood pressure in 12–16-week-old wild type (Wt) and GRAF3 gt/gt mice using radiotelemetry and tail cuff methodology. Both methods revealed a consistent and significant elevation (+20–30 mm Hg) in systolic, diastolic and mean arterial blood pressure in GRAF3 gt/gt mice relative to Wt mice indicating that GRAF3 expression in SMC is required for the maintenance of normal blood pressure ( Fig. 3a , Supplementary Fig. S3a ). Similar circadian variations were in blood pressure were apparent in both lines of mice ( Fig. 3b ). Mice with one copy of the mutant allele (GRAF3 +/gt ) in which vascular GRAF3 mRNA levels were reduced by half also exhibited significant hypertension (+15 mm Hg), indicating that there is a dose-dependent relationship between GRAF3 expression and basal blood pressure ( Supplementary Fig. S3b ). Remarkably, the hypertensive phenotype of GRAF3 gt/gt mice was completely reversed within 90 min after injection of the ROCK inhibitor fasudil (10 mg kg −1 intraperitoneal (i.p. )), which resulted in mean systolic pressures of 81.3 mm Hg versus 79.2 mm Hg in Wt versus GRAF3 gt/gt mice respectively, indicating that elevated RhoA signalling is a major mechanism by which GRAF3 deficiency induces high basal blood pressure. Since elevated RhoA activity is a critical mechanism for the effects of many GPCR-coupled contractile agonists [12] , [14] , we also measured blood pressure by intra-aortic catheterization in animals treated with AngII, ET-1 or PE. As shown in Fig. 3c , agonist-induced increases in systolic blood pressure were significantly enhanced in the GRAF3 gt/gt mice and pretreatment with the ROCK inhibitor, Y27632, completely abrogated the elevated pressor responses strongly supporting increased RhoA activity in this model. 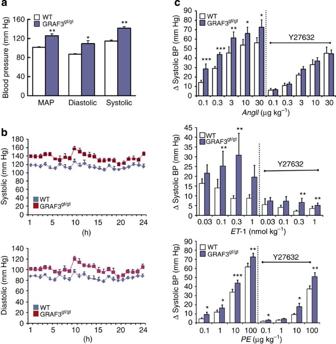Although the effects of GRAF3 depletion on the PE response were less robust, these data are consistent with previous studies suggesting that the pressor effects of PE are less Rho-dependent than AngII and ET-1 (refs 12 , 14 ). Figure 3: GRAF3gt/gtmice exhibit ROCK-dependent hypertension and elevated pressor responses. (a,b) Blood pressures in Wt and GRAF3gt/gtmice were recorded by radiotelemetry over a 24-h period. Measurements from 5-min recordings taken every 30 min were averaged (panela) or plotted as hourly recordings (panelb) (n=5/genotype). Similar values were obtained by standard tail cuff recordings of a separate group of Wt and GRAF3gt/gtmice (seeSupplementary Fig. S3a). (c) Acute arterial pressure was monitored (n=5/genotype) using a Millar catheter prior to and following intravenous injection of indicated vasoconstrictive agent with or without pretreatment of Y27632 (10 mg kg−1i.p.). All values are expressed as means±s.e.m.Pvalues (Student’st-test) are expressed as: *P<0.05; **P<0.01; ***P<0.001. Figure 3: GRAF3 gt/gt mice exhibit ROCK-dependent hypertension and elevated pressor responses. ( a , b ) Blood pressures in Wt and GRAF3 gt/gt mice were recorded by radiotelemetry over a 24-h period. Measurements from 5-min recordings taken every 30 min were averaged (panel a ) or plotted as hourly recordings (panel b ) ( n =5/genotype). Similar values were obtained by standard tail cuff recordings of a separate group of Wt and GRAF3 gt/gt mice (see Supplementary Fig. S3a ). ( c ) Acute arterial pressure was monitored ( n =5/genotype) using a Millar catheter prior to and following intravenous injection of indicated vasoconstrictive agent with or without pretreatment of Y27632 (10 mg kg −1 i.p.). All values are expressed as means±s.e.m. P values (Student’s t -test) are expressed as: * P <0.05; ** P <0.01; *** P <0.001. Full size image Blood pressure is tightly controlled by an integrated signalling balance that involves multiple organs including the heart, brain, kidney and vessel wall. Since the expression of GRAF3 in these organ systems was restricted to the vasculature, we surmised that the hypertensive phenotype in this model was likely due to a RhoA-dependent increase in myogenic tone. However, we first tested the possibility that more common defects in neurogenic or renal hemodynamics were involved. To evaluate sympathetic activity, we measured plasma and urine levels of metanephrine and normetanephrine, the stable metabolites of epinephrine and norepinephrine, respectively. As shown in Supplementary Fig. S3c , we found no significant differences in circulating or excreted catecholamine levels between Wt and GRAF3 gt/gt mice. Accordingly, we observed no significant differences in basal heart rate in GRAF3 gt/gt and Wt mice ( n =5/genotype, mean±s.e.m. of 643.5±36.5 and 666.7±18.7 beats per min, respectively). Moreover, the α 1 -adrenergic blocker, prazosin, caused a similar reduction of blood pressure in Wt and GRAF3 gt/gt mice, and unlike treatment with fasudil, did not normalize the high blood pressure caused by GRAF3 deficiency ( Supplementary Fig. S3d ); indicating that the elevated blood pressure in GRAF3 gt/gt mice was not likely due to enhanced sympathetic stimulation. Kidney structure and function in GRAF3 gt/gt mice was also normal as assessed by a panel of kidney functionality parameters and histological evaluation of periodic acid Schiff and hematoxylin and eosin-stained sections of the renal cortex ( Supplementary Fig. S4a , Supplementary Table S3 ). Notably, urinary albumin (A) and creatinine (CR) levels and A/CR ratios were not significantly different between Wt and GRAF3 gt/gt mice ( Supplementary Fig. S4b ). Thus, we conclude that neuro–renal dysfunction is not likely to play a causative role in the development of hypertension in this model. We next tested whether counterregulatory mechanisms to maintain blood pressure in the face of elevated vessel tone were activated in GRAF3 gt/gt mice. Modulation of angiotensin I-converting enzyme (ACE) levels was an attractive candidate because ACE expression is known to be tightly linked to basal blood pressure. As shown in Supplementary Fig. S4c , we found a significant decrease in ACE protein levels in lungs (the organ in which ACE is most abundant) from GRAF3 gt/gt mice when compared with Wt mice, indicating that negative feedback mechanisms to limit AngII signalling are operative in the GRAF3 gt/gt mice and that the elevated blood pressures observed could be due to a partially compensated increase in Rho-dependent vessel tone. GRAF3 limits RhoA-dependent SMC contractility To further test our hypothesis that GRAF3 depletion induced hypertension by stimulating RhoA-dependent SMC contractility, we next tested the capacity of GRAF3 to stimulate the GTPase activity of RhoA and related small GTPases. To this end, we ectopically expressed full-length Myc-epitope-tagged GRAF3 in COS cells and immunoprecipitated the enzyme using an anti-Myc Ab. Immunoprecipitates were combined with purified His-tagged RhoA, Cdc42, Rac1 and H-Ras and the extent of GTP hydrolysis was measured using a well-characterized method to detect inorganic phosphate. As shown in Supplementary Fig. S5a , immune complexes containing Myc-GRAF3 exhibited a four-fold increase in GAP activity towards RhoA. GRAF3 also induced a modest increase in GAP activity towards Cdc42 but did not promote Rac1 or Ras GTP hydrolysis. We used several gain/loss of function experiments to confirm the ability of GRAF3 to function as a RhoA-GAP in vivo . As shown in Fig. 4a , ectopic expression of GRAF3 in primary vascular SMC markedly attenuated RhoA-dependent actin stress fibre and focal adhesion formation. Conversely, vascular SMC transfected with validated GRAF3 small interfering RNAs exhibited a more contractile morphology that included more abundant focal adhesions increased actin stress fibres, and elevated pMLC ( Fig. 4b,c ). A similar contractile phenotype was observed in vascular SMC isolated from GRAF3 gt/gt mice compared with those isolated from control animals ( Supplementary Fig. S5c ). Importantly, direct measurements of RhoA activity by the GST-rhotekin precipitation assay revealed that activation of RhoA by the lipid agonist, sphingosine-1 phosphate, was significantly elevated and prolonged in GRAF3-depleted SMC when compared with control siRNA-treated cells ( Fig. 4d ). Moreover, using a luminescence-based assay to quantify the GTP-bound form of RhoA, we found that RhoA activity was significantly increased in aortas from GRAF3 gt/gt mice compared with those from Wt mice, validating GRAF3 as a bone fide GAP for RhoA in vivo ( Fig. 5a ). Taken together, these results indicate that GRAF3 plays a major role in limiting RhoA activity in vascular SMC. 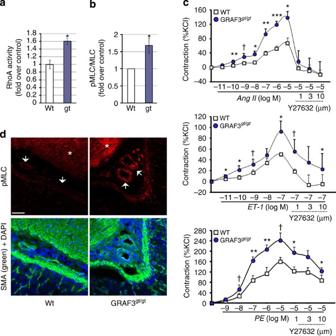Figure 5: GRAF3-depleted vessels exhibit elevated Rho activity and enhanced Rho-dependent contractility. (a) ELISA-based RhoA activity assays were performed on aortic lysates isolated from 6-month-old Wt and GRAF3gt/gtmice (n=6/genotype; mean±s.e.m.;Pvalues (Student’st-test) are expressed as *P<0.05). (b) Densitometric quantification of western blots probed for total- and pMLC in aortas from 6-month-old GRAF3gt/gtversus Wt mice (n=7; mean±s.e.m.;Pvalues (Student’st-test) are expressed as *P<0.05). (c) Dose response of indicated agonist on contraction of aortic segments isolated from Wt and GRAF3gt/gtmice (n=5/genotype). Values (mean±s.e.m.) are expressed as percentage of KCl (124 mM)-induced contraction (no significant difference was observed in maximal contraction of GRAFgt/gtsegments compared with Wt vessels).Pvalues (Student’st-test) are expressed as: †P<0.1; *P<0.05; **P<0.01; ***P<0.001. (d) Immunohistochemistry reveals elevated pMLC levels in vascular SMC in gastric resistance arterioles (arrowheads) and in visceral stomach smooth muscle (asterisk) from GRAF3gt/gtmice. Images are representative of four animals/genotypes. Scale bars, 50 microns. Figure 5: GRAF3-depleted vessels exhibit elevated Rho activity and enhanced Rho-dependent contractility. ( a ) ELISA-based RhoA activity assays were performed on aortic lysates isolated from 6-month-old Wt and GRAF3 gt/gt mice ( n =6/genotype; mean±s.e.m. ; P values (Student’s t -test) are expressed as * P <0.05). ( b ) Densitometric quantification of western blots probed for total- and pMLC in aortas from 6-month-old GRAF3 gt/gt versus Wt mice ( n =7; mean±s.e.m. ; P values (Student’s t -test) are expressed as * P <0.05). ( c ) Dose response of indicated agonist on contraction of aortic segments isolated from Wt and GRAF3 gt/gt mice ( n =5/genotype). Values (mean±s.e.m.) are expressed as percentage of KCl (124 mM)-induced contraction (no significant difference was observed in maximal contraction of GRAF gt/gt segments compared with Wt vessels). P values (Student’s t -test) are expressed as: † P <0.1; * P <0.05; ** P <0.01; *** P <0.001. ( d ) Immunohistochemistry reveals elevated pMLC levels in vascular SMC in gastric resistance arterioles (arrowheads) and in visceral stomach smooth muscle (asterisk) from GRAF3 gt/gt mice. Images are representative of four animals/genotypes. Scale bars, 50 microns. Full size image To provide additional evidence that the hypertensive phenotype observed in GRAF-deficient mice is due to a RhoA-dependent increase in vessel tone, we assessed vasoconstrictor responses in aortic segments isolated from Wt and GRAF gt/gt mice. Similar to our in vivo findings, the constrictor effects of AngII, ET-1 and PE were significantly enhanced in vessel segments from GRAF gt/gt mice, and this enhancement was reversed by Rho-kinase inhibition ( Fig. 5c ). Importantly, both aortic segments and peripheral resistance vessels from GRAF3 gt/gt mice exhibited elevated levels of phosphorylated MLC relative to control mice ( Fig. 5b,d ), supporting the postulate that enhanced RhoA-induced myogenic tone is the main pathogenic factor underlying blood pressure elevation in GRAF3-depleted mice. Our results demonstrate for the first time that GRAF3 regulates blood pressure homoeostasis. Activation of the small GTPase RhoA in vascular SMC has been implicated in the development of vasoconstrictor-induced hypertension [12] , [14] , but until now, the extent that RhoA contributed to the maintenance of basal blood pressure was unknown and the mechanisms that limit RhoA activity in SMC were undetermined. The remarkable SMC-selective expression pattern of this Rho-specific GAP when coupled with the ability of ROCK inhibition to normalize the hypertensive phenotype of GRAF3-deficient animals strongly supports a model in which GRAF3 plays a major role in regulating RhoA-mediated SMC contractility in resistance vessels. Importantly, our results also provide a mechanistic link for the hypertensive locus recently identified within the GRAF3 gene and highlight the need to identify the causal SNPs within this locus and to determine whether these SNPs affect GRAF3 expression in patient populations. Moreover, these findings support the exciting possibility that targeting the induction or activation of GRAF3 may provide a new therapeutic opportunity in the treatment of hypertension. Reagents and tissue samples The anti-Flag (M2), anti-vinculin and SMα-actin antibodies were purchased from Sigma as were the following chemicals: PE, ET-1, AngII and prazosin. ACE and GAPDH antibodies were from Santa Cruz. The myosin light chain2 and phospho-myosin light chain2 (Thr18/Ser19) antibodies were from Cell Signaling. Y27632 was purchased from Calbiochem and sphingosine-1 phosphate (S1P) was from Cayman Chemicals. SM-22 antibody was a generous gift from Mario Gimona. The anti-GRAF1 antibody was described in our previous publication [21] , the GRAF2 antibody was a generous gift from Dr Wen Xiong [23] and a GRAF3 Ab (referred herein as GRAF3Ab1) was purchased from Abnova. The myc-tagged GRAF3 human cDNA clone was purchased from Open Biosystems. GRAF1, GRAF2 cDNAs were previously described [21] , [23] . Human tissue samples were obtained postmortem during autopsy conducted at the University of North Carolina in compliance with current HIPAA rules and regulations. Generation of GRAF3 polyclonal antibody Amino-acid sequences of human, mouse and rat GRAF3 were aligned and the conserved sequence CLSTGRSRKPRGRYTP of GRAF3 was selected for antibody production. Purified peptides were obtained commercially (Invitrogen) and rabbit polyclonal antibodies were generated commercially by standard procedures (Cocalico Biologicals). Sera were screened for immunoreactivity and specificity by western analysis of lysates generated from COS cells transfected with plasmids encoding human GRAF1, mouse GRAF2 or human GRAF3 ( Supplementary Fig. S1 ). Cell culture and transfections Human coronary SMC (huCoSMC; Cambrex) and human aortic SMC (huAoSMC; Cambrex) were maintained in Clonectics SmGM media containing 5% fetal bovine serum, insulin, epidermal growth factor, fibroblast growth factor and gentamicin and were used between passage 3 and 6. Primary aortic vascular SMC were isolated from Wistar rats (RAoSMC) or Wt or GRAF3 gt/gt mice as described [24] . In brief, thoracic aortas were stripped of the endothelial and adventitial layers by microdissection. The SMC in the media were isolated by enzymatic digestion in buffer containing trypsin and collagenase. Cells were maintained in Dulbecco’s modified eagle medium with F12 supplemented with 10% fetal bovine serum and 0.5% penicillin/streptomycin and used from passage 8–16. Each of our preparations is routinely tested for expression of smooth muscle-specific markers (by immunohistochemistry) and the ability to drive smooth muscle-specific expression of reporter constructs. Only the cell lines that are deemed at least 85% pure by these measurements are utilized for further experimentation. Cells were transfected with cDNA constructs using Trans-IT (Mirus) transfection reagents according to manufacturer’s protocol. GRAF3 was depleted from primary aortic SMCs using short interfering RNA (siRNA) (Dharmacon) with the following sequences: sense, 5′-GCCUGAUAGUGACUCCUAUtt-3′; antisense, 5′-AUAGGAGUCACUAUCAGGCtc-3′. Cells were transfected with gene-specific siRNA (100 nmol l −1 ) or non-targeted control siRNA designed against green fluorescent protein using DharmaFECT reagent 1 for 72–96 h. Generation and characterization of GRAF3-deficient mice GRAF3 gene trap ES cells were developed by Genome Research Limited (Sanger Institute, SIGTR ES CE0477) and were distributed by the Mutant Mouse Regional Resource Center at the University of California, Davis. Chimeric mice were produced in-house by injection of GRAF3 +/gt ES cells into the blastocoel cavity of mouse blastocysts by standard procedures. The GRAF3 gt strain was established using three independent chimeras that demonstrated germline transmission when bred to wild-type C57bl6 mice. Homozygous GRAF3 gt / gt mice were generated by crossing F1 GRAF3 gt/+ mice and all experiments were performed using age, sex and littermate genetic controls. For timed pregnancies, day 0.5 of gestation (E0.5) was noon of the day of vaginal plug observation. Genotyping was performed using DNA isolated from tail biopsies using either LacZ (5′-GCATCGAGCTGGGTAATAAGCGTTGGCAAT; 3′-GACACCAGACCAACTGGTAATGGTAGCGAC) or locus-specific primers (5′-TTCGTTGAGACAACTGCACACC; 3′-CCCTTCACACTTTGCTCTCTTAGC). Surgeons were not privy to genotype information. Animal husbandry was provided by staff within the University of North Carolina Division of Laboratory and Animal Medicine and all animal procedures were approved by our accredited American Association for Accreditation of Laboratory Animal Care committee. Blood pressure measurements Conscious blood pressure was measured in male mice aged 12–16 weeks using either radiotelemetry or a tail cuff detection system (Iworx, LabScribe software). For radiotelemetry, implantable mouse BP transmitters (TA11PA-C10, Data Sciences International) were used to record arterial pressure in conscious and freely moving mice (5–6-month-old males weighing 30–35 g). In brief, the mice were anaesthetised with 2% isoflurane, the telemetry catheter was inserted into the left carotid artery of the mouse and the catheter tip was advanced into the thoracic aorta. The catheter was fixed in the left carotid artery and the transmitter was inserted subcutaneously on the backs of mice. Mice were allowed 7 days of recovery following transmitter implantation and were housed individually in a standard polypropylene cage placed on a radio receiver. Mice were maintained in a 12:12-h light–dark cycle. All blood pressure parameters were telemetrically recorded and stored with the Dataquest ART data acquisition system (Data Sciences International). Five-minute recordings were collected every 30 min and data were analysed using Excel software. For the tail cuff measurements, 3–4-month-old male mice were subjected to 20 measurements over a period of 20 min taken every day (between 8:00 and 10:00) for 6 consecutive days as previously described [25] . Data are presented as an average of measurements on the final day. To measure unconscious blood pressure, 6-month-old male mice were anaesthetized with isoflurane, and the right carotid artery was exposed. A pressure transducer (Millar) was inserted through the carotid into the aorta to measure aortic pressure. Vasoconstrictors were administered through a catheter inserted into the left jugular vein. Between doses of vasoactive agents, each animal was allowed to recover its blood pressure to resting levels [25] . In some experiments, Rho-kinase inhibitor (3 or 10 mg kg −1 ) was injected i.p. and pressures were monitored 30 min after dosing. Kidney function measurements Fifty microlitres of urine was collected from 6-month-old male GRAF3 gt/gt and genetic control mice and urinary albumin was determined using an Albuwell-M kit (Exocell, Philadelphia, PA). Spot urine creatinine level was measured on an automated chemical analyser, VT350 from Ortho Clinical Diagnostics. Metanephrine and normetanephrine levels in plasma and urine were measured by ELISA (Metcombi Plasma ELISA, IBL) as per manufacturer’s instructions. Additional kidney panel parameters were analysed in 100 μl blood samples collected from GRAF3 gt/gt and genetic control mice using a VetScan Blood Chemistry Analyser as per manufacturer’s instructions. Myography Two 3-mm aortic segments were collected per mouse (6-month-old males), cleaned from adventitia and placed in ice-cold Krebs buffer (in mmol l −1 ; 120 NaCl, 25 NaHCO 3 , 11 glucose, 1.8 CaCl 2 , 4.7 KCl, 1.2 MgSO 4 , 1.2 KH 2 PO 4 ). The aorta segments were mounted in a Radnoti 4-unit organ bath system (Radnoti Glass Technology) in 20 ml buffer reservoirs containing Krebs (37 °C) aerated constantly with 95% O 2 +5% CO 2 gas mixture. After 45–60 min. stabilization, the baseline tension of the rings was adjusted to 700 mg. All rings were constricted with 124 mM KCl at the end of the experiment and the degree of contraction to indicated agonist was expressed as a percentage of the maximum constriction induced by KCl. LacZ staining and Immunohistochemistry Tissues were processed for LacZ staining using previously published methods [26] . Briefly, tissues were rinsed in 1 × phosphate-buffered saline (PBS) and fixed in 4% paraformaldehyde (PFA)-PBS for 20 min at room temperature. After three 10-min washes in embryo wash buffer (0.1 M phosphate buffer (pH 7.3), 0.1% sodium deoxycholate, 0.02% NP-40, 0.05% bovine serum albumin (Sigma)), tissues were incubated 30 min to overnight at RT in X-Gal staining solution (wash buffer containing 1 mg of X-Gal ml −1 (Sigma), 5 mM ferrocyanide and 5 mM ferricyanide). Tissues were then post fixed in the appropriate fixative, cleared and imaged. For general tissue immunohistochemistry, tissue from mouse pups or patients were harvested, and frozen in OCT or paraffin embedded. Paraffin sections were processed for H&E staining or periodic acid Schiff (PAS) using standardized kits (Sigma). Frozen tissues were sectioned and post fixed with PFA or MeOH using standard conditions and processed for immunohistochemical staining. In brief, sections were permeabilized, blocked and incubated with primary antibodies overnight using the following concentrations: anti-GRAF3 Abs (1:200), α-SMA (1:200), PECAM Ab (1:200), β-GAL (1:200). Cells were processed for immunocytochemistry using previously published methods [24] . In brief, cells were fixed with 4% PFA, permeabilized with 4% Triton X-100 in PBS, incubated with primary antibodies (1:200) for 1 h. After washing with PBS, slides were incubated for 1 h with TRITC or FITC-conjugated goat or rabbit anti-mouse antibodies (2 μg ml −1 ) or Alexa Fluor488- or 555-conjugated phalloidin and 4′,6-diamidino-2-phenylindole (DAPI) to detect filamentous actin and nuclei, respectively. GAP assays COS cells transfected with vector control or Myc-tagged human GRAF3 were lysed in modified RIPA buffer and GRAF3 was immunoprecipitated using a Myc eptitope-specific Ab (2 μg mg −1 lysate). Immunoprecipitates were combined and resuspended in GAP assay buffer and divided accordingly to assess GAP activity towards purified His-tagged RhoA, Rac1, Cdc42 or H-Ras per 500 μg of lysate using the colorimetric-based GTPase activation assay (BK105, Cytoskeleton) as per manufacturer’s instructions. One-half of the amount used in the GAP assay was removed and analysed by immunoblotting to verify the presence of GRAF3 in the experimental but not the negative control samples. Rho activity assays in cultured cells Rat aortic SMC were serum starved overnight prior to treatment with S1P for indicated times. Cell lysates were rotated with 40 μg of a GST-rhotekin Rho binding domain fusion protein immobilized to glutathione-Sepharose 4B beads (Amersham Biosciences) for 15 min at 4 °C in binding buffer (50 mM Tris, pH 7.6, 500 mM NaCl, 0.1% SDS, 0.5% deoxycholate, 1% Triton X-100, 0.5 mM MgCl 2 ) [27] . Beads were precipitated and washed three times (50 mM Tris, pH 7.6, 150 mM NaCl, 1% Triton X-100, 0.5 mM MgCl 2 ) and resuspended in 2 × Laemmli buffer. Proteins were separated on a 15% SDS–PAGE and transferred to 0.2 μm polyvinylidene difluoride (Bio-Rad). After blocking in 3% bovine serum albumin/TBST (20 mM Tris–HCl, 500 mM NaCl, 0.05% Tween-20, pH 7.4) for 30 min at room temperature, blots were probed with 2 μg ml −1 anti-RhoA (26C4) (Santa Cruz Biotechnology) overnight at 4 °C. Loading controls (typically 10%) are taken from each lysate sample prior to pull downs. RhoA activity assays in vessel segments Two-centimeter segments from the descending aorta were collected from Wt and GRAF3 gt/gt mice (6-month-old male and female). The adventitia was rapidly stripped and segments were immediately snap frozen in liquid nitrogen for use in the G-LISA luminescence-based RhoA-specific activation assay (BK121, Cytoskeleton). In brief, frozen aortic segments were crushed using a liquid nitrogen-cooled mortar and pestle and immediately transferred to 200 μl ice-cold lysis buffer containing protease inhibitors (supplied by the manufacturer) followed by sonication (3 × 1-s pulses at 40% power; Sonics VibraCell). Lysates were clarified by centrifugation (2 min at 4 °C) and the level of RhoA activity was measured in 20-μg samples as per the manufacturer’s instructions (Cytoskeleton). Western blotting To examine protein levels, lysates from cells or tissues were prepared by lysing in a modified RIPA buffer with protease and phosphatase inhibitors [24] . Protein concentration was determined by using a colorimetric BCA assay (Pierce). Lysates were electrophoresed on 10–15% SDS–polyacrylamide gel, transferred to nitrocellulose and immunoblotted with specific antibodies as indicated using a 1:1000 dilution. Blots were washed in TBST (TBS plus 0.05% Triton X), followed by incubation with either horseradish peroxidase conjugated-rabbit anti-mouse antibody or—protein A sepharose (Amersham) at a 1/2,000 dilution. Blots were visualized after incubation with chemiluminscence reagents (ECL, Amersham). Semi quantitative RT–PCR Cells or organs harvested from mice were homogenized, and RNA was extracted using Zymo or Qiagen RNA isolation kit. Semi quantitative RT–PCR was performed with the following primers: GRAF3 exons 1–4, 5′-CTGCCCACTCTGGAGTTCAGCG, 3′-GCTGCACCGATCTGTTCTTTTCG; GRAF3 exons 10-17, 5′-GAACCGATTTACACGTTACCCG, 3′-GGTTGGACCAAATATGACACCG; GAPDH 5′-ATGGGTGTGAACCACGAGAA, 3′-GGCATGGACTGTGGTCATGA. Statistical analysis All data representt least three separate experiments presented as means±s.e.m. Means were compared by Student’s t- test or analysis of variance (where indicated) and statistical significant is reported as P values. All other data, including western blot analysis and RT–PCR, are representative of at least three individual experiments and band intensities were quantified using ImageJ software. Sample sizes were chosen based on an extensive literature search and standard exclusion criterion of two s.d. from the mean were applied. How to cite this article: Bai, X. et al. The smooth muscle-selective RhoGAP GRAF3 is a critical regulator of vascular tone and hypertension. Nat. Commun. 4:2910 doi: 10.1038/ncomms3910 (2013).